Optimization of non-periodic plasmonic light-trapping layers for thin-film solar cells Non-periodic arrangements of nanoscale light scatterers allow for the realization of extremely effective broadband light-trapping layers for solar cells. However, their optimization is challenging given the massive number of degrees of freedom. Brute-force, full-field electromagnetic simulations are computationally too time intensive to identify high-performance solutions in a vast design space. Here we illustrate how a semi-analytical model can be used to quickly identify promising non-periodic spatial arrangements of nanoscale scatterers. This model only requires basic knowledge of the scattering behaviour of a chosen nanostructure and the waveguiding properties of the semiconductor layer in a cell. Due to its simplicity, it provides new intuition into the ideal amount of disorder in high-performance light-trapping layers. Using simulations and experiments, we demonstrate that arrays of nanometallic stripes featuring a limited amount of disorder, for example, following a quasi-periodic or Fibonacci sequence, can substantially enhance solar absorption over perfectly periodic and random arrays. The rapid advances in the fields of nanophotonics and plasmonics [1] are spurring a wave of new research aimed at improving the performance of thin-film solar cells [2] . From this work, it is becoming apparent that nanoscale light-trapping structures have the potential to outperform conventional macroscopic surface textures that are commonly applied on thick crystalline solar cells. However, the design and optimization of the ideal nanophotonic light-trapping layers is currently under active debate. Whereas the ray-optics theory of light trapping was of great value in designing conventional thick cells [3] , [4] , [5] , it was recently pointed out that this theory breaks down for ultra-thin cells and absorption enhancements can potentially exceed the well-known Yablonovitch limit [6] , [7] . This limit states that absorption enhancement in a medium with a refractive index n cannot exceed a factor of 4 n 2 /sin 2 θ , where θ is the half-angle of the emission cone in the medium surrounding the cell [8] . Meanwhile, significant developments are also taking place in the inexpensive production of ultra-thin semiconductor layers via epitaxial lift-off and wafer splicing technologies that can significantly reduce consumption of expensive semiconductor material [9] , [10] . With the advances in nanotechnology, it is also plausible that in the future the ideal light-trapping layers can be made in a scalable fashion [11] , [12] . For fundamental and practical reasons, it is thus worth developing rapid optimization schemes for light-trapping layers based on wave-optics that are effective in the limit of ultra-thin cells for which the thickness is less than the absorption depth of sunlight. In this work, we demonstrate the significant benefits of engineering non-periodic particle arrangements for broadband light trapping in ultra-thin solar cells. This builds on the many excellent optimization studies of light-trapping layers using periodic particle arrangements. The importance of some amount of disorder in textured surfaces has a recognized beneficial effect in photovoltaic cells. Many effective fabrication routes for light-trapping layers involve annealing, etching or self-assembly steps that naturally result in some randomness. There are an increasing number of excellent efforts on the development of smart algorithms for the design of metallic nanostructure arrays that afford broadband light concentration [13] . In addition, there has been excellent work aimed at analysing the effect of randomness in surface textures on the performance of solar cells [14] , [15] , [16] , [17] . That said, there is no systematic and general strategy currently available to optimize the degree and type of disorder in light-trapping layers. Such a strategy would ideally suggest the best light-trapping structures, their geometry and spatial arrangement on a cell. Brute-force, full-field electromagnetic simulations are unfortunately computationally too time intensive to identify high-performance solutions in a vast design space. For this reason, we develop a semi-analytical light-trapping model that allows for a more rapid optimization and a deeper understanding why some non-periodic arrays outperform others. We illustrate its usefulness with ultra-thin Si cells decorated with non-periodic, metallic stripe arrays. 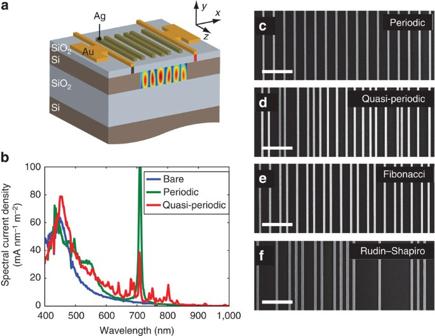Figure 1: Optimized non-periodic stripe arrays. The non-periodic arrays facilitate enhanced light trapping in ultra-thin semiconductor layers. (a) A schematic of the silicon-on-insulator (SOI) photodetector structure decorated with a quasi-periodic stripe array. (b) Simulated spectral short-circuit current density for the device with a periodic (green) and a quasi-periodic (red) array of Ag stripes. The blue curve shows the simulated response for a reference device with a bare 50 nm thick Si layer and 20 nm thick SiO2layer on top. (c–f) SEM images of fabricated devices featuring (c) periodic, (d) quasi-periodic, (e) Fibonacci and (f) Rudin–Shapiro arrays of Ag stripes. The scale bar, 1 μm. Performance of non-periodic light-trapping layers Figure 1a schematically shows how the light-trapping performance of different non-periodic light-trapping layers on ultra-thin crystalline Si films can be quantified and compared. Light-trapping layers of interest are first fabricated on high-quality, commercially available silicon-on-insulator wafers. When the resulting structures are top-illuminated with sunlight, photocarriers are produced in the thin Si layer. These carriers can be extracted via laterally spaced contacts. Photocurrent measurements taken at different illumination wavelengths and polarizations of light facilitate a quantitative assessment of the spectral light-trapping properties of a light-trapping structure of interest [18] . Figure 1: Optimized non-periodic stripe arrays. The non-periodic arrays facilitate enhanced light trapping in ultra-thin semiconductor layers. ( a ) A schematic of the silicon-on-insulator (SOI) photodetector structure decorated with a quasi-periodic stripe array. ( b ) Simulated spectral short-circuit current density for the device with a periodic (green) and a quasi-periodic (red) array of Ag stripes. The blue curve shows the simulated response for a reference device with a bare 50 nm thick Si layer and 20 nm thick SiO 2 layer on top. ( c – f ) SEM images of fabricated devices featuring ( c ) periodic, ( d ) quasi-periodic, ( e ) Fibonacci and ( f ) Rudin–Shapiro arrays of Ag stripes. The scale bar, 1 μm. Full size image In optimizing the metallic nanostructure arrays, one typically aims to boost light absorption by taking advantage of the high near-fields surrounding metallic structures when excited close to their surface plasmon resonance frequency and effective light trapping in the active semiconductor by coupling to waveguide modes supported by the solar cell [19] . Significant attention has been devoted to the optimization of the metal nanostructure size and shape [2] , [20] , [21] , [22] , [23] , [24] . It was found that relatively large (50–150 nm) metallic particles are desirable because they exhibit relatively little absorption losses due to a favourable ratio of the scattering to absorption cross section. In this work, we will employ optimized metallic stripes and direct our attention to optimizing their spatial arrangement to enhance coupling to waveguided modes. This strategy is of value as the coupling to waveguide modes for most realistic cells designs provides the largest absorption enhancements. Even for unique cases where absorption enhancements related to high near-fields are significant, they tend to be very similar for different non-periodic and periodic arrays with a similar average stripe spacing ( Supplementary Note 2 ). We start with a quantitative example that illustrates the benefits of introducing non-periodic features in a light-trapping layer. Figure 1b shows the simulated spectral short-circuit current densities from a 50 nm Si film decorated with either a periodic (green) or a quasi-periodic (red) array of 60 nm wide Ag stripes (See Methods and Fig. 1a ). In these simulations, we illuminated the structure at normal incidence with randomly polarized sunlight (standard AM 1.5G spectrum) and assumed a 100% internal quantum efficiency for the devices. For the periodic array, we chose a stripe-spacing of 290 nm as this spacing produced the highest possible short-circuit current according to our simulations. Next, the quasi-periodic array was produced by randomly displacing the stripes of the periodic array with a Gaussian distribution in the displacements. The response of the bare Si film is also shown for reference (blue). The photocurrent spectrum under standard AM 1.5G solar illumination of the bare Si film features the highest photocurrents on the short wavelength side due to stronger Si absorption well above the bandgap. The changes in the spectral response obtained with the periodic stripe array can be understood by viewing the array as a grating. This grating efficiently couples the incident light to a waveguide mode supported by the Si slab when the reciprocal lattice vector of the grating matches to the propagation constant of the guided mode. The coupling to both transverse magnetic (TM) modes with H-field pointed along the stripes and transverse electric (TE) waveguide modes increases the path length of sunlight in the Si and enhances absorption. The sharp increase in the short-circuit current at 710 nm is due to such a coupling resonance. A broader peak near the surface plasmon resonance of an individual Ag stripe is also seen at 550 nm. The sharp features weaken in the case of the quasi-periodic array and an increased broadband enhancement is obtained in return. This is expected as the multiple periods present in the spatial Fourier transform of the quasi-periodic grating enable effective coupling at many wavelengths. By integrating the spectral photocurrent we find that the periodic array gives rise to a 40% increase in the photocurrent over the bare Si film. The non-periodic array does even better and provides an enhancement of 55%. At this point, it is clear that a qualitative understanding can be obtained about the features in the spectrum and a quantitative increase can be realized with the non-periodic structure. However, there is no clear understanding on how one should go about systematically optimizing the non-periodic spatial arrangement of the stripes. Semi-analytical model for optimizing the non-periodicity In the following, we aim to describe our semi-analytical model, which can be applied to quickly identify promising non-periodic spatial arrangements of the stripes that maximize the absorption of sunlight in the Si layer. From the outset, it is unclear what average stripe spacing would be ideal and what degree and type of disorder are needed. Whereas a perfectly periodic structure appears not to be ideal, a perfectly random structure may not be good either. A perfectly random structure exhibits a spectrally flat coupling response and may efficiently couple light into the cell in a spectral region that lies outside the solar spectrum or below the semiconductor bandgap. Based on Parseval’s theorem known from applied mathematics [25] , it is impossible to increase the coupling efficiency at all wavelengths. Thus an enhanced coupling efficiency at some frequencies will come at the cost of a reduced efficiency at other frequencies. As a result, a perfectly random grating is bound to exhibit a less-than-optimal efficiency by ‘wasting’ coupling strength in more-or-less useless parts of the electromagnetic spectrum. The mentioned semi-analytical model was developed to rapidly calculate the absorption spectrum for any non-periodic light-trapping array. This enables one to quickly identify high-performance light-trapping arrays and to gain an understanding of why some light-trapping layers outperform others. For example, it provides insight into the question why Fibonacci ( Fig. 1e ) and quasi-periodic arrays with a limited amount of disorder can outperform perfectly periodic ( Fig. 1c ) and virtually random Rudin Shapiro [26] ( Fig. 1f ) arrays. The model, which is detailed and verified in Supplementary Note 1 , only requires knowledge of the light-scattering properties of the array elements (metallic stripes in our case) and the optical behaviour of the waveguide modes supported by the solar cell. As such, it can enable a significantly faster exploration of the phase space of possible spatial arrangements of light-trapping elements than full-field simulations. 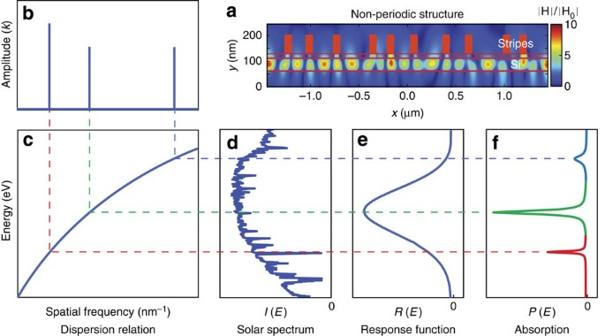Figure 2: Semi-analytical model for calculating absorption spectra. This figure demonstrates the semi-analytical model used for calculating the absorption spectrum of a non-periodic grating structure. (a) Full-field simulation of the fields in a non-periodic grating structure. (b) Spatial Fourier transform of the non-periodic grating. (c) Dispersion diagram for a selected waveguided mode supported by the solar cell. (d) Solar spectrum. (e) Response function as determined by the solar cell and scattering particles. (f) The absorption spectrum. Figure 2 provides a graphic explanation of the essential features of our semi-analytical model and compares it with a full-field simulation approach. Figure 2a shows an example of a full-field simulation of a non-periodic array of Ag stripes placed on top of a thin Si layer. Although such simulations can be used to determine the light absorption in the semiconductor layer, they are computationally expensive and do not allow for a rapid array optimization. Alternatively, we can start by identifying the spatial frequencies K present in the non-periodic array. This is accomplished by taking a spatial Fourier transform of the grating structure consisting of a series of delta functions sitting at the centre of each of the scattering stripes. As illustrated above for the periodic and quasi-periodic arrays, these spatial frequencies determine at which illumination wavelengths coupling of sunlight will occur. In this tutorial example, we find three dominant spatial frequencies whose location and Fourier amplitudes A K are represented by the blue bars in Fig. 2b . Next, we can determine at which optical frequencies (that is, wavelengths) sunlight can strongly couple to the waveguide modes supported by the cell by plotting their dispersion relations. For simplicity, we only consider the coupling to one specific mode in this example. Later this procedure is generalized to treat multi-mode solar cells. Figure 2c shows graphically that the dispersion relation uniquely links each spatial frequency present in the grating to a specific optical frequency at which a coupling resonance occurs. The actual absorption at each of the coupling resonances is of course dependent on the solar intensity I S at each of the coupling resonance frequencies ( Fig. 2d ) and on the solar cell’s ability to capitalize on these coupling resonances. This ability is quantified by an optical response function R ( ω ) that captures the frequency-dependent response of the solar cell structure to the presence of the stripe-grating ( Fig. 2e ). This function is dependent on the scattering properties of the stripe and the properties of the waveguided modes supported by the solar cell. These properties are easily determined from a full-field electromagnetic simulation that is significantly simpler and computationally less expensive than large area simulation of a realistic non-periodic light-trapping structure consisting of many elements (see Supplementary Note 1 ). The total absorption for a realistic cell that supports multiple modes can now be expressed as: Figure 2: Semi-analytical model for calculating absorption spectra. This figure demonstrates the semi-analytical model used for calculating the absorption spectrum of a non-periodic grating structure. ( a ) Full-field simulation of the fields in a non-periodic grating structure. ( b ) Spatial Fourier transform of the non-periodic grating. ( c ) Dispersion diagram for a selected waveguided mode supported by the solar cell. ( d ) Solar spectrum. ( e ) Response function as determined by the solar cell and scattering particles. ( f ) The absorption spectrum. Full size image Here, contributions to the total absorption are summed for all resonances, each resonance having a frequency ω i,K results from one spatial frequency K of the grating that facilitates coupling to one of the waveguides modes i . A K is the spectral weight of the grating at the Fourier coefficient K . For very thin solar cells that only support one mode that significantly contributes to the absorption of sunlight, the subscript i can be dropped. In Supplementary Note 1 it is shown that γ i is a coefficient that quantifies the coupling of sunlight via a stripe to a waveguide mode i . The magnitude of the coefficients and quantify the attenuation per unit length of the associated propagating waves in the semiconductor layer due to intrinsic absorption and scattering into radiation modes, respectively. In this expression, is the group velocity of the mode. The magnitudes of these quantities are all frequency dependent and together they determine the spectral shape of the response function. Finally, D is the average distance between the particles in the array. This equation is consistent with the expression of total absorption by Yu et al. [6] However, the expression for the total absorption in this form highlights the separate contributions of the grating and scatterer and thus provides a powerful and practical way to optimize performance in actual solar cell absorbers. Below, we will use this formula as a guide to understand why some non-periodic grating structures outperform others in enhancing solar cell efficiency. It should be noted that equation (1) can be used to calculate the absorbed power at a target frequency of interest by summing the contributions of relevant coupling resonances. If one is interested in calculating and optimizing the absorbed solar flux, one simply needs to replace the solar intensity I S by the solar flux F S in this equation. Figure 2f shows the absorption spectrum with three peaks whose spectral position is directly determined by the spatial frequencies in the grating and the dispersion relation of the considered waveguide mode. It is worth noting that the calculated absorption spectra do not have sharp features like the spatial Fourier spectra of the array. This results from the fact that each coupling resonance is broadened owing to various loss mechanisms (absorption, scattering) in the waveguide coupling and propagation (see Supplementary Note 2 ). 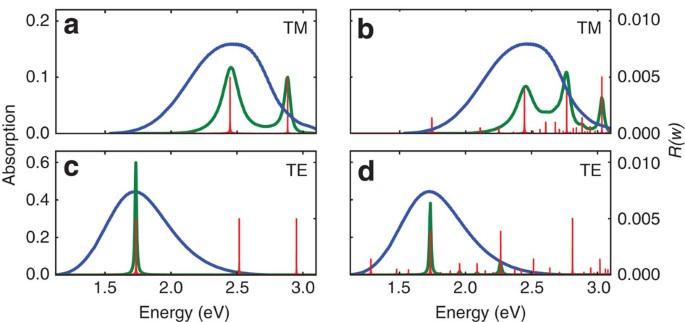Figure 3: Optimization strategy for non-periodic light-trapping structures. Plot of the response function (blue) and absorption spectra (green) as calculated for a periodic (a,c) and Fibonacci (b,d) array of Ag stripes placed on a 50 nm Si film. Both the case for TM (a,b) and TE (c,d) polarizations are shown. For reference, the magnitudes of the Fourier amplitudesAKfor the periodic and Fibonacci arrays are also plotted as red vertical lines at the photon energies where they induce coupling. Application of the model to calculate absorption spectra Figure 3 shows the calculated absorption spectra for realistic structures consisting of an ultra-thin (50 nm) Si film decorated with a periodic (a,c) grating and a grating following a Fibonacci sequence (b,d). The spectra were produced by following the approach described above. The procedure for realizing gratings following a Fibonacci or other non-periodic sequence is explained in Supplementary Note 3 . The film is sufficiently thin so that the light absorption is dominated by a single-optical mode, simplifying the analysis and discussion. For illustration purposes, we also start by assuming an idealized flat illumination spectrum ( F s ( ω )=constant) instead of the real solar spectrum, which exhibits many sharply peaked features that tend to obscure some of the essential physics. For a real solar cell optimization, we will later numerically maximize the overall absorbed flux using the AM 1.5G spectrum. For randomly polarized sunlight, we also need to consider the cell response to light with a TM and TE polarization, with the electric field normal or along the stripes, respectively. Figure 3: Optimization strategy for non-periodic light-trapping structures. Plot of the response function (blue) and absorption spectra (green) as calculated for a periodic ( a , c ) and Fibonacci ( b , d ) array of Ag stripes placed on a 50 nm Si film. Both the case for TM ( a , b ) and TE ( c , d ) polarizations are shown. For reference, the magnitudes of the Fourier amplitudes A K for the periodic and Fibonacci arrays are also plotted as red vertical lines at the photon energies where they induce coupling. Full size image The red vertical lines in the four panels of Fig. 3 represent the location and magnitude of spatial frequencies A K for the two arrays. Whereas the periodic array displays just two lines in the spectral range where the response function is large, the Fibonacci sequence shows a large number of lines with a reduced magnitude. The blue and green curves represent the response curves and calculated absorption spectra, respectively. The strength of absorption in the spectra is given in terms of the ratio of absorbed flux in the Si layer and the incident solar flux. It can be seen that the response curves for TE and TM polarizations are both quite broad, reflecting the broad absorption spectrum of Si and the efficient coupling to the relevant mode over a broad range of frequencies. Their spectral shape and location are quite different as these two polarizations induce a very different scattering response from the stripes and couple to different modes of the Si slab. For example, the TM response curve is shifted significantly to higher energies due to the surface plasmon resonance of the Ag stripes near 2.5 eV. The period for the periodic stripe array was chosen to be 290 nm, which after a quick optimization with our semi-analytic model was found to maximize the overall absorbed photon flux. For the flat illumination spectrum, maximizing the absorbed flux translates into maximizing the sum of the products R K ( ω ) for all K . Physically, this corresponds to maximizing the coupling where the response function is large. In this case, the optimization resulted in one spatial frequency close to the maximum of the response function (see Fig. 3a ). Figure 3b shows for the Fibonacci array with the same average stripe spacing. This array generates more spatial frequencies in the region where the response function is larger for both the TE and TM polarizations. For this reason, a higher overall absorption can be expected. However, at the cost of introducing new resonances, the strength of the coupling resonances ( ) tends to be smaller than for the periodic grating as we are spreading the coupling power over more spatial frequencies. To determine which structure is best, we analyse the predicted absorption spectra and find that the total, integrated absorbed flux for the Fibonacci array shows an increase of 15% over the periodic array. It is important to note that the calculation of these absorption spectra is extremely quick after the response function is determined. For this reason, many different non-periodic structures can be quickly tested or inverse problems can be defined to rapidly identify high-performance solutions. Supplementary Note 2 provides several examples of other non-periodic, high- and low-performance structures. Understanding the critical role of the response function Previous optimization studies on periodic light-trapping structures have greatly benefitted from the generation of absorption enhancement maps. Such maps plot the absorption enhancement in the semiconductor layer that results from the presence of a stripe array versus the incident energy E and a reciprocal characteristic spacing G =2 π / D (refs 19 , 22 , 27 ). Here, we again generate such E–G maps to further illustrate how the optimized Fibonacci array outperforms the optimized periodic array. 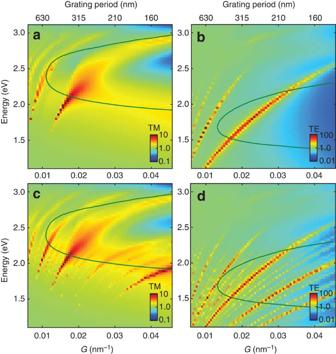Figure 4: Effects of disorder on the performance of a light-trapping layer. (a) Map of the absorption enhancements in a 50 nm thick Si film versus the incident photon energy and inverse period of the periodic stripe-array for TM illumination. (b) Similar map for the periodic array but now for TE illumination. (c) Similar map for the Fibonacci sequence under TM illumination. (d) Similar map for the Fibonacci sequence under TE illumination. All of the colour bars are on a logarithmic scale to the base 10. Note the different scale for the TE and TM maps chosen based on the fact that the features in the TE maps tend to be larger in magnitude (but narrower in width). The green curve separates out those spectral regions where the response function is high and waveguide coupling leads to significant contributions to the absorption of sunlight. Figure 4a–d shows absorption enhancement maps for periodic and Fibonacci arrays under TM and TE illumination. Each point in these maps is obtained from a full-field simulation on a solar cell. For the Fibonacci pattern, we define D as the average separation between stripes to allow a simple comparison with the periodic array for which we take D equal to the period. The maps exhibit two distinct features that can be correlated with large enhancements. The relatively dispersionless (that is, flat), broad yellow bands around 2 eV in the two TM maps result from an effective excitation of the surface resonance of an individual stripe. Their occurrence is not associated with a specific array configuration and is primarily related to the stripe geometry and dielectric environment. A slight redshift is observed with increasing G (that is, decreasing D ) because of the increased coupling between stripes. The sharper, dispersive features in these maps are related to effective coupling to waveguide modes. To analyse the possible contributions of the various coupling resonances to the total amount of absorbed sunlight, we also outline the spectral region where the response function is large—somewhat arbitrarily chosen as 7% of the total absorption in the bare Si film—by a green curve. We will term this region the absorption band (AB). The contributions of the resonances get larger inside the AB up to ~20% of the total absorption in the bare Si film. Large absorption enhancements found outside of the AB may look exciting at first, but do not provide substantive contributions to the overall absorption. Figure 4: Effects of disorder on the performance of a light-trapping layer. ( a ) Map of the absorption enhancements in a 50 nm thick Si film versus the incident photon energy and inverse period of the periodic stripe-array for TM illumination. ( b ) Similar map for the periodic array but now for TE illumination. ( c ) Similar map for the Fibonacci sequence under TM illumination. ( d ) Similar map for the Fibonacci sequence under TE illumination. All of the colour bars are on a logarithmic scale to the base 10. Note the different scale for the TE and TM maps chosen based on the fact that the features in the TE maps tend to be larger in magnitude (but narrower in width). The green curve separates out those spectral regions where the response function is high and waveguide coupling leads to significant contributions to the absorption of sunlight. Full size image From these maps, it is clear that for both the periodic and Fibonacci arrays the average spacing of 290 nm ( G ~0.02 nm −1 ) indeed makes an excellent choice as it places several good absorption enhancement features within the AB. The maps also show that larger stripe spacings tend to produce less and less absorption related to waveguide coupling, consistent with the 1/ D 2 scaling in equation (1). Smaller stripe spacings tend to pull large enhancement features out of the desirable spectral region where the response function is large. As such, there is an optimum spacing that maximizes the overall absorption. It is clear that the Fibonacci array features more strong resonances within the AB than the periodic one for both TM and TE polarization. This is desirable when broadband absorption for randomly polarized sunlight needs to be optimized. If this is the target, optimized non-periodic structures always outperform the periodic ones as they offer more flexibility to generate spatial frequencies that facilitate coupling in the AB for both TE and TM polarization. For periodic structures a chosen period that optimizes absorption for one polarization often results in a non-optimized situation for the other polarization. In Supplementary Note 2 , we analysed a variety of non-periodic structures and show that too much randomness can be detrimental. For example, we find that virtually random patterns such as arrays following the Rudin–Shapiro sequence exhibit fewer high-strength (that is, large spatial frequencies within the AB and the overall absorption is reduced. From the above discussion, it is clear that the spectral response function has a critical role in indentifying the high-performance light-trapping solutions. Experimental verification of the semi-analytic model The usefulness and validity of the presented analytical model was tested by using it to identify optimized periodic, Fibonacci, quasi-periodic and Rudin–Shapiro light-trapping arrays for thin Si layers. These arrays were chosen as they feature varying degrees of disorder. Scanning electron microscopy images of the fabricated arrays are shown in Fig. 1c–f . High-performance arrays could rapidly be identified by maximizing the integrated absorption for AM 1.5G illumination using our semi-analytic model, without the need for time-consuming full-field simulations of the complex devices. To verify that the optimized arrays indeed can give rise to enhanced light absorption, we performed both spectral photocurrent measurements and full-field simulations on the optimized devices, as shown schematically in Fig.1a (see Methods). 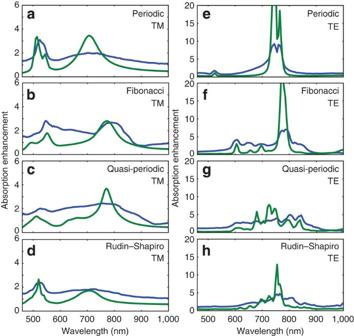Figure 5: Photocurrent enhancement spectra for various degrees of disorder. Photocurrent spectra obtained by experiment (blue) and full-field electromagnetic simulations (green) for Si layers decorated with Ag stripe arrays with (a) periodic, (b) Fibonacci, (c) quasi-periodic and (d) Rudin–Shapiro patterns for (a–d) TM and (e–h) TE polarizations. The simulated TE and TM enhancements were divided by a factor 2 in order to more easily compare the simulated peak positions with the experimental ones. Figure 5a–h shows experimental photocurrent enhancement spectra for TM and TE polarizations on all of the arrays. The enhancement in photocurrent was determined with respect to a bare Si structure and thus provides a direct measure of the absorption enhancement due to presence of the arrays. Full-field electromagnetic simulations of the predicted photocurrent enhancement are also shown for the same structures. It can be seen that both the full-field simulations and the experiments exhibit significant, broadband photocurrent enhancements for all of the investigated arrays. The predicted peak positions in the simulated photocurrent spectra nicely correspond to the locations found in the experiments and clearly demonstrate the presence and importance of tunable coupling resonances in enhancing the photocurrent. This point underscores the usefulness of the proposed optimization strategy aimed at strategically placing coupling resonances across the solar spectrum, with a fast semi-analytical technique. The experimentally measured absorption enhancement peaks were found to be broadened and reduced in magnitude compared with those predicted by full-field simulations. These discrepancies between experiment and theory were found to be similar for all array structures and can be explained by a combination of factors, including a previously observed and quantified reduction in the conductivity of the nanoscale Ag stripes versus bulk Ag by a factor of 2–3 ( [18] ), roughness of the surface of the stripes, and deviations from the targeted stripe widths and spacings. The integrated photocurrent enhancements were 148% for the periodic array, 161% for Fibonacci, 178% for quasi-periodic and 145% for Rudin–Shapiro patterns. In agreement with our prediction, the periodic and virtually random structures performed poorest, whereas the Fibonacci and quasi-periodic arrays that exhibit the best coupling, where the response function is large, performed best. Figure 5: Photocurrent enhancement spectra for various degrees of disorder. Photocurrent spectra obtained by experiment (blue) and full-field electromagnetic simulations (green) for Si layers decorated with Ag stripe arrays with ( a ) periodic, ( b ) Fibonacci, ( c ) quasi-periodic and ( d ) Rudin–Shapiro patterns for ( a – d ) TM and ( e – h ) TE polarizations. The simulated TE and TM enhancements were divided by a factor 2 in order to more easily compare the simulated peak positions with the experimental ones. Full size image With the presented semi-analytical mode, the challenge of optimizing absorption of sunlight in an ultra-thin solar cell has been translated into the significantly simpler challenge of identifying a non-periodic array of scatterers that exhibit effective optical coupling in a spectral region where the sun emits light and the spectral response function of a cell is large. It also provides new insights in the important question why certain non-periodic arrays of scatterers perform better than periodic or perfectly random arrays. It is clear that both the spacing and spatial arrangement of the particles is important in optimizing the overall absorption of sunlight. As such, this work provides a conceptual framework that furthers our understanding of complex non-periodic nanophotonic systems and assists in the development of robust optimization strategies for light-trapping coatings using, for example, genetic engineering or inverse problems. Full-field simulations on non-periodic arrays To rapidly identify optimum non-periodic light-trapping layers, we developed a semi-analytic light-trapping model that is detailed in Supplementary Notes 1–2 and verified by full-field electromagnetic simulations. The model was tested in simulations and experiments on various periodic and non-periodic arrays consisting of 60 nm wide and 70 nm thick Ag stripes placed on a 50 nm thick Si layer. A 20 nm thick thermal oxide was used to space the metal stripes from the Si layer to avoid significant damping of the surface plasmon resonance of the stripes [19] . In the simulations, the optical properties of Ag are taken from experimental data [28] . Sample fabrication Schottky barrier photodetectors as shown in Fig. 1 a were realized in the 50-nm thick Si layer of a lightly doped (1 ohm cm) n-type silicon-on-insulator wafer using standard photolithography techniques. The electrical contacts of the detector were spaced by 120 μm. Between the contacts, we generated arrays of Ag stripes with periodic, Fibonacci, quasi-periodic and Rudin–Shapiro patterns using standard electron-beam lithography, metal deposition and lift-off techniques. Photocurrent measurements were carried out using a Fianium supercontinuum white-light source coupled to a Spectra Physics monochromator. The photocurrent signal was measured using a Keithley SourceMeter connected to a SRS lock-in amplifier. The 40 × 40 μm 2 stripe arrays were illuminated with a Gaussian beam using a 5 × Mitutoyo objective providing a spot size of 10 μm diameter. How to cite this article: Pala, R. A. et al. Optimization of non-periodic plasmonic light-trapping layers for thin-film solar cells. Nat. Commun. 4:2095 doi: 10.1038/ncomms3095 (2013).